Hour-glass magnetic excitations induced by nanoscopic phase separation in cobalt oxides The magnetic excitations in the cuprate superconductors might be essential for an understanding of high-temperature superconductivity. In these cuprate superconductors the magnetic excitation spectrum resembles an hour-glass and certain resonant magnetic excitations within are believed to be connected to the pairing mechanism, which is corroborated by the observation of a universal linear scaling of superconducting gap and magnetic resonance energy. So far, charge stripes are widely believed to be involved in the physics of hour-glass spectra. Here we study an isostructural cobaltate that also exhibits an hour-glass magnetic spectrum. Instead of the expected charge stripe order we observe nano phase separation and unravel a microscopically split origin of hour-glass spectra on the nano scale pointing to a connection between the magnetic resonance peak and the spin gap originating in islands of the antiferromagnetic parent insulator. Our findings open new ways to theories of magnetic excitations and superconductivity in cuprate superconductors. The spin excitations in high-temperature superconducting (HTSC) cuprates with a quasi two-dimensional layered crystal structure resemble an hour-glass if plotted as a function of energy and momentum transfer [1] , [2] , [3] , [4] , [5] , [6] , [7] , [8] , [9] , [10] , [11] , [12] , [13] . Understanding the mechanism of these magnetic excitations and their relation to high-temperature superconductivity remains one of the great challenges in condensed matter physics. Therefore, the recent discovery of such excitation spectra in an isostructural but insulating cobaltate reference system La 5/3 Sr 1/3 CoO 4 has attracted enormous attention [12] . The assumed presence of charge stripes in this cobalt oxide pointed to the presence of (fluctuating) stripes in the isostructural cuprates [12] and, hence, suggested the importance of charge stripes for the physics in the high-temperature superconductors. In charge stripe phases the doped charges (holes) segregate into stripes, whereas antiferromagnetism is able to recover in the charge-depleted regions between these stripes. However, the very recent finding of an hour-glass dispersion in a checkerboard charge ordered cobaltate La 1.6 Sr 0.4 CoO 4 has shown that hour-glass spectra are not necessarily connected to charge stripe phases [13] . La 5/3 Sr 1/3 CoO 4 is a compound with a hole-concentration even further from half-doping that exhibits diagonal magnetic satellite reflections around third-integer positions in reciprocal space. For this hole-doping the isostructural nickelates that also exhibit diagonal magnetic satellites at the same positions in reciprocal space exhibit the most stable diagonal charge stripe order. Hence, also for La 5/3 Sr 1/3 CoO 4 the incommensurate magnetic peaks have been interpreted within a charge stripe scenario [12] , [14] . Here we demonstrate that there are no signatures of charge stripes in La 5/3 Sr 1/3 CoO 4 . Instead, we observe a fractal microstructure with a nanoscopic distribution of undoped and hole-doped regions indicating that hour-glass spectra consist of excitations with distinct origin on the nanometer scale. Whereas the low-energy regime is still dominated by excitations within the nano-sized hole-doped regions, at highest energies only the nanoscopic undoped islands can be excited. In our nanoscale phase separation scenario the energy of the neck of the hour-glass could be interpreted as the spin-gap within undoped islands of type of the antiferromagnetic parent insulator La 2 CoO 4 . Hard X-ray diffraction measurements Using 100 keV hard X-rays at the synchrotron we first studied the charge correlations in La 5/3 Sr 1/3 CoO 4 . In a disordered charge stripe scenario the corresponding charge stripe ordering superstructure reflections should exhibit similar peak widths as the magnetic reflections [15] . However, in our highly precise synchrotron measurements we were not able to detect any indications for charge stripe ordering reflections (for L =0 and L =3>>0) in La 5/3 Sr 1/3 CoO 4 with an unprecedented accuracy of about 10 −9 of a strong Bragg reflection, see Fig. 1a,b . A charge stripe-ordered La 5/3 Sr 1/3 NiO 4 reference sample with same hole-concentration exhibits strong charge stripe ordering peaks in both equivalent scans. Note that the huge Co 2+ ions and the small Co 3+ ions exhibit distinctly bigger differences in their ionic radii than the corresponding Ni ions [16] such that any occurring stripe phases should be much easier to detect in cobaltates than in nickelates. Furthermore, magnetic stripes and charge stripes can not be decoupled due to the nonmagnetic properties of the Co 3+ ions [17] , [18] and due to the highly insulating localized nature [18] of this cobaltate system. Instead of charge stripe ordering reflections we, surprisingly, observe weak checkerboard charge ordering intensities at half-integer H and K positions in reciprocal space that survive up to room temperature, see Fig. 1c,d . This important finding indicates that the robust checkerboard charge ordering correlations still persist also far away from half-doping down to one-third doping in the La 2− x Sr x CoO 4 system and that there are no disordered charge stripe phases in this entire incommensurate magnetic regime of the La 2− x Sr x CoO 4 system (1/3≤ x <1/2). Instead, checkerboard charge ordered regions with roughly 0.7(2) nm correlation length appear. The remaining Co 2+ ions have to be distributed somewhere into the cobalt oxygen planes as the hole-doping in La 5/3 Sr 1/3 CoO 4 is far below half-doping. Hence, checkerboard charge ordered regions have to be interspersed with La 2 CoO 4 -like undoped islands within a nano-phase separation scenario. 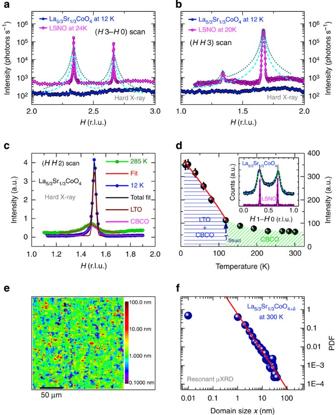Figure 1: Charge correlations Synchrotron radiation single-crystal X-ray diffraction measurements using 100 keV hard X-rays at beamline P07 at PETRA III. (a) Measured intensities of scans along (H3−H0) andbscans along (H H3) for La5/3Sr1/3CoO4and a roughly one-third hole-doped LSNO reference sample. Strong fundamental Bragg reflections are of the order of 1010photons/s. Intensities ina,bhave been normalized to the monitor (incident beam) for a comparison of cobaltate and nickelate reference sample. The dashed lines are Lorentzian peaks with same integrated intensity as for the charge stripe ordering peaks of the LSNO reference sample but with peak widths that have been multiplied by the width ratio of the incommensurate magnetic peaks of both compounds measured with neutrons (inset ofd); dotted lines are additionally normalized to the (200) peak intensities. No diagonal charge stripe correlations like in the nickelates could be observed for La5/3Sr1/3CoO4. (c) Weak checkerboard charge ordering reflections appear at half-integer positions for even values ofLalready at room-temperature. The correlation length that could be obtained from Lorentzian fits indicates an average nanometer size of checkerboard charge ordered regions (~0.7(2) nm). Below the structural transition tetragonal→orthorhombic additional sharp octahedral tilting reflections appear on top of the broad checkerboard charge ordering reflections. (d) The temperature dependence of the total integrated intensities at half-integer peak positions. The inset shows neutron scans across the magnetic satellites for La5/3Sr1/3CoO4and ~1/3 hole-doped LSNO. (e) Spatial map of the checkerboard charge ordered domain size distribution on the crystal surface along theab-direction obtained from μXRD measurements at beamline P10 at PETRA-III. The distribution appears to be inhomogeneous and checkerboard charge-ordered regions with varying domain size can be observed. (f) The PDF36of the checkerboard charge ordered domain size along theab-direction. The behaviour of the PDF tail obeys a perfect power-law (PDF(x)=x−α) indicating a scale-free distribution in the checkerboard charge ordered domain sizes, thus corroborating our nano-phase-separation scenario. Only ~1% (~11%) of the measured sample exhibits domain sizes bigger than 50 (10) unit cells. Error bars are s.d. Figure 1: Charge correlations Synchrotron radiation single-crystal X-ray diffraction measurements using 100 keV hard X-rays at beamline P07 at PETRA III. ( a ) Measured intensities of scans along ( H 3− H 0) and b scans along ( H H 3) for La 5/3 Sr 1/3 CoO 4 and a roughly one-third hole-doped LSNO reference sample. Strong fundamental Bragg reflections are of the order of 10 10 photons/s. Intensities in a , b have been normalized to the monitor (incident beam) for a comparison of cobaltate and nickelate reference sample. The dashed lines are Lorentzian peaks with same integrated intensity as for the charge stripe ordering peaks of the LSNO reference sample but with peak widths that have been multiplied by the width ratio of the incommensurate magnetic peaks of both compounds measured with neutrons (inset of d ); dotted lines are additionally normalized to the (200) peak intensities. No diagonal charge stripe correlations like in the nickelates could be observed for La 5/3 Sr 1/3 CoO 4 . ( c ) Weak checkerboard charge ordering reflections appear at half-integer positions for even values of L already at room-temperature. The correlation length that could be obtained from Lorentzian fits indicates an average nanometer size of checkerboard charge ordered regions (~0.7(2) nm). Below the structural transition tetragonal→orthorhombic additional sharp octahedral tilting reflections appear on top of the broad checkerboard charge ordering reflections. ( d ) The temperature dependence of the total integrated intensities at half-integer peak positions. The inset shows neutron scans across the magnetic satellites for La 5/3 Sr 1/3 CoO 4 and ~1/3 hole-doped LSNO. ( e ) Spatial map of the checkerboard charge ordered domain size distribution on the crystal surface along the ab -direction obtained from μXRD measurements at beamline P10 at PETRA-III. The distribution appears to be inhomogeneous and checkerboard charge-ordered regions with varying domain size can be observed. ( f ) The PDF [36] of the checkerboard charge ordered domain size along the ab -direction. The behaviour of the PDF tail obeys a perfect power-law (PDF( x )= x − α ) indicating a scale-free distribution in the checkerboard charge ordered domain sizes, thus corroborating our nano-phase-separation scenario. Only ~1% (~11%) of the measured sample exhibits domain sizes bigger than 50 (10) unit cells. Error bars are s.d. Full size image Resonant micro X-ray diffraction measurements We analysed the real-space distribution of the charge correlations in La 5/3 Sr 1/3 CoO 4 by means of resonant scanning micro X-ray diffraction (μXRD) measurements. The μ XRD technique has been already successfully applied for the study of phase separation in the isostructural cuprates [19] , [20] . Here, we additionally applied an incident X-ray energy of 7,719 eV to measure any Co 2+ /Co 3+ charge ordering correlations in resonance for a high contrast of charge ordering reflections. Moving the sample under a 2 μm focussed beam with an x-y translator, we scanned a sample area of 202 × 210 μm 2 collecting 10,605 different diffraction patterns at ~300 K. For each scanned point of the sample the (0.5 0.5 2) peak profile has been extracted and the full-width half-maximum (FWHM) along ab -direction has been evaluated to obtain the domain size of the checkerboard charge ordered regions. The spatial map of this domain size along ab -direction is shown in Fig. 1e . To quantify [21] the distribution of undoped islands and checkerboard charge ordered regions, we calculated the probability density function (PDF) of the measured domain sizes, see Fig. 1f . Similar to that observed in the isostructural cuprates [19] , [20] for oxygen ordering superstructure reflections, the PDF tail presents a perfect power-law behaviour and can be fitted by the function PDF( x )= x − α , where x is the ab -domain size of checkerboard charge ordering and α =1.99(8) is the critical exponent of the power-law. This particular behaviour highlights a scale-free distribution of the checkerboard charge ordered domain size in La 5/3 Sr 1/3 CoO 4 . From the non power-law region of the PDF we can estimate the expected values of the checkerboard charge ordering ab -domain size that amounts to ~0.8(2) nm. Thus, our μXRD measurements indicate a fractal microstructure up to a maximum observed domain size of ~39 nm and corroborate the presence of a disordered checkerboard charge ordered phase interspersed with undoped islands and, hence, our nano phase separation scenario. Neutron scattering measurements Studying the magnetic excitations in La 5/3 Sr 1/3 CoO 4 in detail, we surprisingly observe a hitherto unknown high-energy magnon band above the entire classical hour-glass dispersion, see Fig. 2a . The polarization analysis confirms that this additional high-energy mode is magnetic in origin. Note that this is the first observation of an additional separated high-energy magnon band appearing completely above an entire hour-glass dispersion. Usually, one expects optical modes in a magnon dispersion without hour-glass shape or the optical magnon mode merges with the low-energy dispersion such that both together are forming an hour-glass-shaped dispersion [22] , [23] , [24] . Also a 40% Sr-doped cobaltate within the checkerboard charge ordered regime exhibits this same additional high-energy mode, see Fig. 2c . Our polarized neutron measurements uncover the interesting nature of these magnetic excitations, whereas all low-energy spin excitations within the entire classical hour-glass dispersion are mainly in-plane excitations (see Fig. 2b ), the additional yet unknown high-energy mode appears to be an out-of-plane polarized magnon band, see Fig. 2a . As the low-energy excitations in La 5/3 Sr 1/3 CoO 4 basically resemble on the excitations in the half-doped cobaltate La 1.5 Sr 0.5 CoO 4 and as the high-energy excitations resemble on the excitations of the undoped parent compound La 2 CoO 4 including the out-of-plane polarized additional high-energy mode, our observations suggest that the hour-glass dispersion is not one single dispersion, but, that it consists of two dispersions with distinct origin, see Fig. 3 . The first dispersion arises from the low-energy magnetic excitations of the hole-doped regions that are governed by frustration and that exhibit chiral or non-collinear magnetic phases and the second one arises from the high-energy magnetic excitations of the undoped islands strongly resembling on the dispersion of the undoped parent compound (La 2 CoO 4 ) that exhibits a spin gap and an additional high-energy magnon mode. This model is shown schematically in Fig. 3 . The intensity enhancement at the magnon merging point or neck of the hour-glass (we would like to call this by definition also simply resonance peak for the non-superconducting cobaltates throughout this article) that can be traced with energy scans at the planar antiferromagnetic (AFM) wavevector exhibits a surprisingly similar energy dependence like in equivalent scans for La 2 CoO 4 , see Fig. 2a (dark yellow dots). This clearly points to a related origin of this resonance peak energy in La 5/3 Sr 1/3 CoO 4 and the spin gap in La 2 CoO 4 . This is also consistent with the temperature dependence of this energy scan and a beginning of a closing of this spin gap with increasing temperature, see Fig. 4a and also compare ref. 25 for the temperature dependence of the long-range ordered undoped compound La 2 CoO 4 (with higher magnetic ordering temperature). In contrast the high-energy part of the hour-glass-shaped dispersion in La 5/3 Sr 1/3 CoO 4 does not exceed to exactly that high energies as the dispersion for pure La 2 CoO 4 . This might be owed to the structural changes and the amount of disorder in the charge sector with extremely short-ranged La 2 CoO 4 -like correlations. However, this difference in the maximum energy clearly proves that we did not simply measure the magnetic signal of a macroscopically phase-separated sample with conventional phase separation. Our polarized neutron study underlines our findings as the hitherto unknown high-energy magnon band clearly belongs to an out-of-plane excitation, whereas the outwards dispersing contributions from the neck of the hour-glass are mostly in-plane excitations, see Fig. 2d , and, thus, fully compatible to the La 2 CoO 4 excitation spectrum [25] . Also the 40% Sr-doped cobaltate exhibits qualitatively the same energy scan at the planar AFM wavevector, see Fig. 2c . This is fully in agreement with our scenario that the spin gap within the undoped islands is responsible for the resonance-like increase of intensity at the neck of the hour-glass, as the spin anisotropy gap energy should be much less doping dependent than a dispersion that starts from different incommensurate magnetic peak positions in samples with different hole-doping. Also the comparison of magnetic intensities of high and low energy magnetic signal for two different hole-concentrations corroborates our whole scenario, as the additional high energy mode is the strongest for low Sr-doping where larger fractions of undoped regimes can be expected, compare Fig. 2e,f . Furthermore, the temperature dependence of the hour-glass dispersion is also consistent with our nano phase separation model, see Fig. 4 . The temperature dependence of the high energy excitations is different from the strongly temperature affected low energy part. Fitting the magnetic peaks of the constant-E scans at 5 meV and at 29 meV (shown in Fig. 4b,c ) with two symmetric gaussians indicates a different temperature dependence in both energy regions. In our model, this could be explained by a different decrease of the spin wave stiffness of upper and lower dispersions with rising temperature, see Fig. 4d . Furthermore, the peak widths are unchanged with temperature, see inset in Fig. 4d . This unaffected peak width reflects an almost temperature independent dynamic correlation length. In our nano phase separation model this would be naturally implied by the limiting factor of the limited static domain size of hole-doped checkerboard charge ordered and undoped islands. For the low-energy excitations this dynamic correlation length would be of the order of ~0.6 nm that would nicely correspond to the measured average correlation length of the static checkerboard charge order which amounts to ~0.7 nm. 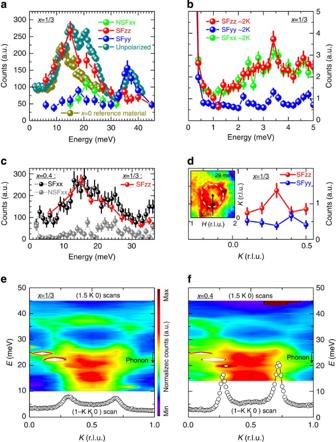Figure 2: Spin excitations (a) Energy scans at the planar AFM wavevector studied by polarized neutrons. In-plane polarized excitations that can be detected in the Spin-Flip (SF) channel ||z(z⊥scattering plane) emerge at the neck of the hour-glass (red data points). Surprisingly, an additional high-energy mode appears at elevated energies. The polarization analysis indicates the out-of-plane character of these high-energy excitations as it can be detected in the SF channel ||y(blue data points;ywithin scattering plane,y⊥Q). In addition, also the results of unpolarized neutron scattering experiments of La5/3Sr1/3CoO4measured at the IN8 spectrometer (dark cyan data points) and La2CoO4taken from ref.25(dark yellow data points) are shown. As can be seen, the small additional 20 meV feature belongs to a phonon, whereas the resonance-like increase of intensity is located ~15 meV that is close to the in-plane anisotropy gap of La2CoO4. (b) Study of the nature of the low-energy excitations by polarized neutrons measured by constant-Qscans at (1/2−ε1/2+ε0) at ~2 K at the IN12 spectrometer. The in-plane character of these low-energy magnetic excitations is revealed. (c) Also La1.6Sr0.4CoO4exhibits the same energy scan at the planar AFM wavevector measured with polarized neutrons in the channel ||Qthat detects in-plane and out-of-plane excitations simultaneously. (d) For the outwards dispersing branches above the neck of the hour-glass also in-plane excitations can be detected in the SF channel ||z. The inset shows the corresponding scan in reciprocal space within a 29 meV constant-E map. (e,f) Comparison of strength of the high-energy magnetic intensities for different Sr-doping measured at the IN8 spectrometer. Intensities have been normalized to the Phonon peak intensity (black arrrow). Intensity error bars are statistical error bars calculated by the square root of intensity. Figure 2: Spin excitations ( a ) Energy scans at the planar AFM wavevector studied by polarized neutrons. In-plane polarized excitations that can be detected in the Spin-Flip (SF) channel || z ( z ⊥ scattering plane) emerge at the neck of the hour-glass (red data points). Surprisingly, an additional high-energy mode appears at elevated energies. The polarization analysis indicates the out-of-plane character of these high-energy excitations as it can be detected in the SF channel || y (blue data points; y within scattering plane, y ⊥ Q ). In addition, also the results of unpolarized neutron scattering experiments of La 5/3 Sr 1/3 CoO 4 measured at the IN8 spectrometer (dark cyan data points) and La 2 CoO 4 taken from ref. 25 (dark yellow data points) are shown. As can be seen, the small additional 20 meV feature belongs to a phonon, whereas the resonance-like increase of intensity is located ~15 meV that is close to the in-plane anisotropy gap of La 2 CoO 4 . ( b ) Study of the nature of the low-energy excitations by polarized neutrons measured by constant- Q scans at (1/2− ε 1/2+ ε 0) at ~2 K at the IN12 spectrometer. The in-plane character of these low-energy magnetic excitations is revealed. ( c ) Also La 1.6 Sr 0.4 CoO 4 exhibits the same energy scan at the planar AFM wavevector measured with polarized neutrons in the channel || Q that detects in-plane and out-of-plane excitations simultaneously. ( d ) For the outwards dispersing branches above the neck of the hour-glass also in-plane excitations can be detected in the SF channel || z . The inset shows the corresponding scan in reciprocal space within a 29 meV constant-E map. ( e , f ) Comparison of strength of the high-energy magnetic intensities for different Sr-doping measured at the IN8 spectrometer. Intensities have been normalized to the Phonon peak intensity (black arrrow). Intensity error bars are statistical error bars calculated by the square root of intensity. 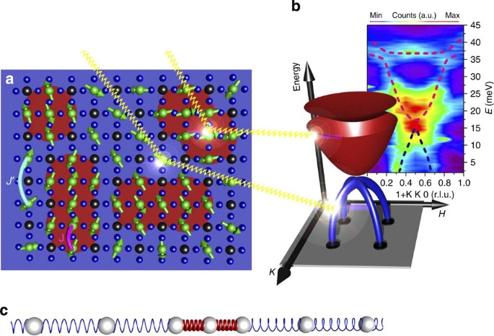Figure 3: The two hour-glass dispersions (a) Our nano-phase separation model within La5/3Sr1/3CoO4. The doping of additional electrons or Co2+ions (green spheres) at Co3+sites (black spheres) of an ideal checkerboard charge ordered structure of the half-doped AFM parent compound induces strong frustration as we already pointed out in ref.13. However, due to the large ratio of the exchange interactionsJ/J′ the non-collinearity of the spin structure can be expected basically in the hole-doped regions (blue) and not within the undoped islands (red) where the spins should be aligned in a much more collinear manner. Neutrons (yellow waves) scattered from these different regions will behave differently. (b) Schematic presentation of the magnetic spectra in La2−xSrxCoO4together with measured neutron scattering intensity behind. The blue contributions indicate the low-energy excitations originating from the hole-doped regions (blue areas ina) with smallJ,′ whereas the high-energy signal arises from excitations within the undoped regions (red areas ina) with largeJ. Here, the upper dispersion (red) is shifted somewhat to higher energies such that the lower dispersion (blue) becomes clearly visible, although both dispersions should inter-penetrate each other. The yellow waves indicate neutrons that were either scattered from the undoped islands or from the hole-doped regions. (c) One-dimensional mechanical analogy of decoupled oscillations of balls within a one-dimensional chain that are connected with weak (blue) or strong (red) force constants. Full size image Figure 3: The two hour-glass dispersions ( a ) Our nano-phase separation model within La 5/3 Sr 1/3 CoO 4 . The doping of additional electrons or Co 2+ ions (green spheres) at Co 3+ sites (black spheres) of an ideal checkerboard charge ordered structure of the half-doped AFM parent compound induces strong frustration as we already pointed out in ref. 13 . However, due to the large ratio of the exchange interactions J / J ′ the non-collinearity of the spin structure can be expected basically in the hole-doped regions (blue) and not within the undoped islands (red) where the spins should be aligned in a much more collinear manner. Neutrons (yellow waves) scattered from these different regions will behave differently. ( b ) Schematic presentation of the magnetic spectra in La 2− x Sr x CoO 4 together with measured neutron scattering intensity behind. The blue contributions indicate the low-energy excitations originating from the hole-doped regions (blue areas in a ) with small J ,′ whereas the high-energy signal arises from excitations within the undoped regions (red areas in a ) with large J . Here, the upper dispersion (red) is shifted somewhat to higher energies such that the lower dispersion (blue) becomes clearly visible, although both dispersions should inter-penetrate each other. The yellow waves indicate neutrons that were either scattered from the undoped islands or from the hole-doped regions. ( c ) One-dimensional mechanical analogy of decoupled oscillations of balls within a one-dimensional chain that are connected with weak (blue) or strong (red) force constants. 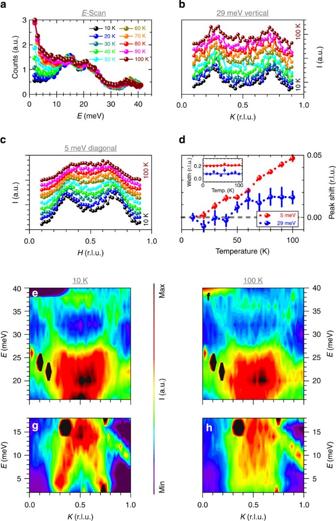Figure 4: Temperature dependence of the hour-glass dispersion (a) The temperature dependence of energy scans at the planar AFM wavevector. (b) Temperature dependence of constant-Escans at 29 meV scanning vertical through the planar AFM wavevector. (c) Temperature dependence of constant-E scans at 5 meV scanning diagonal through the magnetic satellite positions. (d) Temperature dependence of the magnetic peak positions relative to the peak positions at lowest temperature (10 K) if two Gaussians are fitted to the data inb,c. The inset shows the corresponding peak widths. (e–h) Colour-contour plots of neutron scattering intensity measured as a function of energy and momentum transfer for low (10 K:e,g) and higher temperatures (100 K:f,h). This temperature dependence is consistent with our nano phase separation model (see text). Intensities inb–hare multiplied by. Error bars are s.d. (obtained from gaussian fits). Intensity error bars are statistical error bars calculated by the square root of intensity. Full size image Figure 4: Temperature dependence of the hour-glass dispersion ( a ) The temperature dependence of energy scans at the planar AFM wavevector. ( b ) Temperature dependence of constant- E scans at 29 meV scanning vertical through the planar AFM wavevector. ( c ) Temperature dependence of constant-E scans at 5 meV scanning diagonal through the magnetic satellite positions. ( d ) Temperature dependence of the magnetic peak positions relative to the peak positions at lowest temperature (10 K) if two Gaussians are fitted to the data in b , c . The inset shows the corresponding peak widths. ( e – h ) Colour-contour plots of neutron scattering intensity measured as a function of energy and momentum transfer for low (10 K: e , g ) and higher temperatures (100 K: f , h ). This temperature dependence is consistent with our nano phase separation model (see text). Intensities in b – h are multiplied by . Error bars are s.d. (obtained from gaussian fits). Intensity error bars are statistical error bars calculated by the square root of intensity. Full size image The physical reason for the occurrence of these two distinct sets of dispersions that we schematically present in Fig. 3b can be understood as well. The magnetic exchange interaction J ′ between two Co 2+ ions in the hole-doped (checkerboard charge ordered) regions is much smaller than the comparably large magnetic interactions J within the undoped islands of La 2 CoO 4 type ( J >> J ′), see Fig. 3a . Thus, the excitations within the hole-doped regions stay at low energies, whereas the excitations of the undoped islands (red area in Fig. 3a ) exceed to high energies. The reason that the excitations within both types of regions are that strongly de-coupled is the huge difference in the exchange couplings J and J ′ that is of the order of ~9.7 and ~1.4 meV, respectively [17] , [25] , and also the existence of a sizeable spin gap within the phase with larger J . For a simplified mechanical analogy see Fig. 3c . The neck of the hour-glass dispersion results basically from the existence of a spin gap within the undoped islands. Note that such a spin gap of these dimensions has been observed in La 2 CoO 4 (ref. 25 ), see Fig. 2a (dark yellow dots). Our spin wave calculations based on our nano-phase separation scenario, which we modelled with Monte Carlo simulations using the Metropolis algorithm, are able to reproduce all basic features of the hour-glass dispersion including our additional high-energy mode and, thus, corroborate our experimentally found nano phase separation model, see Methods section and Fig. 5 . First of all, chiral or non-collinear magnetic structures arise due to frustration in analogy to a proposed scenario for LSCO [26] , [27] . More important, our calculations are able to reproduce the surprising additional high-energy mode that arises from out-of-plane excitations exactly as observed in our polarized neutron scattering experiments (see also the movie in the Supplementary Material ). Furthermore, our simulations indicate—in close relation to our mechanical analogy shown in Fig. 3c —that the hole-doped (checkerboard charge ordered) regions can be only excited at lower energies, whereas at high energies only the undoped islands of type of the antiferromagnetic parent insulator La 2 CoO 4 can be excited, see Fig. 5 . Hence, our spin wave simulations corroborate our experimental finding of a microscopically split origin of upper and lower part of magnetic excitations within the so-called hour-glass dispersion. 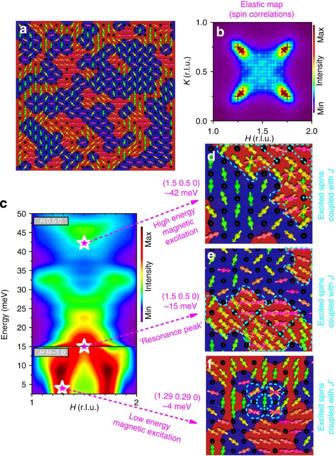Figure 5: Spin wave simulations (a) Spin correlations within a 30 × 30 lattice calculated for our nano phase separation model. A non-collinear magnetic structure arises from frustration. Black spheres: nonmagnetic Co3+ions, coloured spheres: Co2+ions, red shaded areas: undoped islands (Co2+ions coupled with at least oneJ), blue shaded areas: checkerboard charge ordered islands (Co2+ions coupled only withJ′). The direction of spins is additionally indicated by a colour coding. (b) Fourier transformation of the non-excited spin configurations in Q-space. The vertical crosses indicate wavevectors expected for an ideal checkerboard charge ordered system and the diagonal crosses indicate the expected incommensurate magnetic peak positions for our nominal hole-concentration according to an experimentally observed linear hole-doping dependence13. (c) Simulated spin excitation spectrum. The basic features of the hour-glass dispersion can be reproduced. (d–f) Calculated magnetic excitations. The movement of the spins is indicated by plotting strongest displacements of the spins for this spin excitation on top of the static spin configuration such that direction and colour of that spin are differing when spins are involved in the excitation. In addition, the dashed cyan lines mark regions of excited spins. Our theoretical simulations yield a purely out-of-plane character of the novel high-energy spin excitations, see also ourSupplementary Video File; (here ind, the out-of-plane oscillation has been artificially transformed into an in-plane excitation). As can be seen, the checkerboard charge ordered regions (coupled withJ′≪J) can be excited only at low energies, whereas at high energies only the undoped islands (coupled withJ>>J′) can be excited. At the crossing of the hour-glass the undoped islands become in resonance—hence the occurrence of a resonant peak—and exhibit the strongest movements. Figure 5: Spin wave simulations ( a ) Spin correlations within a 30 × 30 lattice calculated for our nano phase separation model. A non-collinear magnetic structure arises from frustration. Black spheres: nonmagnetic Co 3+ ions, coloured spheres: Co 2+ ions, red shaded areas: undoped islands (Co 2+ ions coupled with at least one J ), blue shaded areas: checkerboard charge ordered islands (Co 2+ ions coupled only with J ′). The direction of spins is additionally indicated by a colour coding. ( b ) Fourier transformation of the non-excited spin configurations in Q-space. The vertical crosses indicate wavevectors expected for an ideal checkerboard charge ordered system and the diagonal crosses indicate the expected incommensurate magnetic peak positions for our nominal hole-concentration according to an experimentally observed linear hole-doping dependence [13] . ( c ) Simulated spin excitation spectrum. The basic features of the hour-glass dispersion can be reproduced. ( d – f ) Calculated magnetic excitations. The movement of the spins is indicated by plotting strongest displacements of the spins for this spin excitation on top of the static spin configuration such that direction and colour of that spin are differing when spins are involved in the excitation. In addition, the dashed cyan lines mark regions of excited spins. Our theoretical simulations yield a purely out-of-plane character of the novel high-energy spin excitations, see also our Supplementary Video File ; (here in d , the out-of-plane oscillation has been artificially transformed into an in-plane excitation). As can be seen, the checkerboard charge ordered regions (coupled with J ′ ≪ J ) can be excited only at low energies, whereas at high energies only the undoped islands (coupled with J >> J ′) can be excited. At the crossing of the hour-glass the undoped islands become in resonance—hence the occurrence of a resonant peak—and exhibit the strongest movements. Full size image Finally, the insulating cobaltates appear to be a copper-free reference system that enables us to understand some most basic underlying mechanisms of hour-glass spectra and that overcomes the obstacle of fluctuating charges, thus unraveling a direct connection between the occurrence of hour-glass magnetic spectra and nano phase separated microstructures. Our findings might help to understand the observations of isotropic high-energy magnetic excitations in the isostructural La 2− x Sr x CuO 4 (LSCO) materials [7] , [11] , [28] or the recent observations of similar high-energy magnetic excitations in superconducting LSCO samples and the undoped parent materials probed by resonant inelastic X-ray scattering (RIXS) [29] , [30] . Whereas it seems to be reasonable to attribute the spin gap within the undoped islands of the cobaltates to an anisotropy gap like in La 2 CoO 4 (ref. 25 ), in the cuprates the higher energy scales within the excitation spectra would suggest a different physics. Spin gaps with higher energies are known for singlet-triplet excitations of cuprate materials due to finite size effects of the undoped regions [31] , [32] , [33] , [34] . Crystal synthesis A.C.K. has grown the La 2− x Sr x CoO 4 and La 2− x Sr x NiO 4 (LSNO) single crystals by the optical floating zone technique using a CSC four-mirror image furnace following the route described in ref. 13 . The crystals are single phase as ascertained by high-resolution powder X-ray diffraction measurements. The single crystals are single domain as ascertained by Laue X-ray and single crystal neutron diffraction techniques. Owing to the measured incommensurability in these neutron measurements the oxygen content in La 5/3 Sr 1/3 CoO 4+ δ is close to stoichiometric δ ~0.01. The crystal quality was further ascertained by WDX measurements indicating close to nominal stoichiometry within our single crystals La 1.675(6) Sr 0.325(2) CoO 4+ δ (averaged over 10 measurements). Finally, we performed a highly accurate single crystal X-ray diffraction measurement at a Bruker D8 VENTURE single-crystal X-ray diffractometer equiped with a Photon large area CMOS detector. The sample has a spherical shape with 95(5) μm diameter. In total, 93,028 reflections have been collected using Mo K α radiation and a bent graphite monochromator for ~3 times intensity enhancement. The internal R -value amounts to 2.20% with a redundancy of 50.4. The R and weighted R -value in the refinement on F 2 amount to 1.66 and 4.19% and the goodness of fit amounts to 1.27. The resulting structural parameters within space group I4/mmm are z (La/Sr)=0.362234(1), U iso (La/Sr)=0.005885(2), U iso (Co)=0.004560(4), U iso (O1)=0.009831(25), z (O2)=0.173122(24), U iso (O2)=0.020418(36), a =3.8552(3) Å, c =12.6267(9) Å, and the refinement of the Sr-occupancy indicates that x amounts to 33.2(2)% that is close to stoichiometric. The nominally 40% Sr doped reference sample was already described in ref. 13 and has a composition of La 1.591(3) Sr 0.404(1) CoO 4.01(1) according to ICP-OES and titration measurements. Z.W.L. has also grown another La 5/3 Sr 1/3 CoO 4+ δ single crystal following the route described in ref. 12 , which reveals larger additional oxygen contents than the sample grown by the author A.C.K. and was only used for the measurement of the temperature dependence of the magnetic excitations and the μXRD experiments. Comparing the magnetic incommensurabilities the excess of oxygen amounts to δ =0.035(1) in this sample. However, the dispersion matches reasonably well with that of ref. 12 , thus indicating a similar incommensurability. Complementary inductively coupled plasma optical emission spectroscopy (ICP-OES) and WDX measurements indicate close to nominal stoichiometry of that sample La 1.675(11) Sr 0.326(3) CoO 4+ δ and La 1.663(7) Sr 0.330(6) CoO 4+ δ , respectively. Synchrotron measurements The synchrotron radiation single crystal X-ray diffraction measurements have been performed at beamline P07 at PETRA III at DESY using 100 keV hard X-rays monochromatized by a bent Si(111) double monochromator providing an energy resolution of 0.2%. The signal was analyzed with a Si-Ge(111) gradient crystal analyser and detected with a point detector. The measured samples were very ~(0.5–1.5) 3 mm 3 sized single crystals. The monitor-normalized (200) reflection intensities of La 5/3 Sr 1/3 CoO 4 and the LSNO reference sample amount to 2.7 × 10 10 photons s −1 and 9.7 × 10 9 photons s −1 . The μXRD experiments were carried out at the Coherence Beamline P10 at PETRA III. The X-ray beam is monochromatized using a cryogenically cooled Si(111) double crystal monochromator. An X-ray energy of 7,719 eV with a bandwidth of dE / E ~1.4·10 −4 was selected. About 1 m upstream of the focusing optics situated at 85.6 m from the undulator source a slit of a size of 150 × 75 μm 2 selected a highly coherent fraction of the X-ray beam. This collimated coherent X-ray beam was focused using the in-vacuum Beryllium compound refractive lens (CRL) transfocator of the P10 beamline to a size of about 2 × 2 μm 2 at the sample position 2.2 m downstream of the transfocator centre. A pair of JJ X-ray in-vacuum slits located at 220 and 800 mm upstream of the sample was used to clean up the small angle scattering signal of the CRL’s from focused X-ray beam. The incident flux on the sample was about 1–2 × 10 11 photons s −1 . The scattered signal from the sample was recorded at a sample to detector distance of 25 cm using a Pilatus 300 K detector. Neutron scattering measurements For the elastic and inelastic neutron scattering experiments one large La 5/3 Sr 1/3 CoO 4 , La 1.6 Sr 0.4 CoO 4 or LSNO single crystal has been mounted with an [100]/[010] orientation in the scattering plane. The inelastic neutron scattering experiments at the 1T.1 and 2T spectrometers have been performed in constant- k f operation mode with fixed focusing pyrolytic graphite (PG) monochromator and analyser using two PG filters for the suppression of higher order contamination. At the IN8 spectrometer an experimental set-up with double focusing PG monochromator and analyzer as well as two PG filters was used. At the IN22 spectrometer a set-up with fixed vertically focusing (125 cm radius) and flat horizontal (111) Heusler monochromator and vertically focusing and flat horizontal (111) Heusler analyser was used. For polarization analysis a CRYOPAD polarimeter for spherical polarization analysis was installed. The flipping ratio amounts to ~16. A PG filter was used for suppression of higher order contamination. At the IN12 spectrometer that is situated at the end of a horizontal elliptic focusing guide a double focusing PG monochromator and a horizontally focusing Heusler analyser were used. The incident neutron beam was polarised with a polarising cavity. For polarization analysis a set-up with Helmholtz coils for linear polarization analysis was installed. The flipping ratio amounts to ~17.4. A velocity selector was used for elimination of higher order contributions (suppression better than 10 −4 ). The temperature dependence of the magnetic excitations in La 5/3 Sr 1/3 CoO 4+ δ was measured at the PUMA spectrometer using a double focusing PG monochromator and analyser as well as two PG filters for elimination of higher order contamination. Numerical simulations The Monte-Carlo simulations for simulating disordered checkerboard charge ordered structures are based on the Metropolis algorithm similar as in ref. 15 . Only one potential for Coulomb repulsion and another for steric repulsion of two adjacent Co 2+ ions with large ionic radii has been considered for our simulation of the charge distribution on a N × N lattice ( N =30, 50) and statistical/random distribution of the charges at each site with a certain probability (here 40%) in the initial step for about a dozen configurations. To model the magnetism we introduce AFM exchange interactions between the Co 2+ ions i , j with spin operators and , respectively (the Co 3+ ions were treated as nonmagnetic): . According to our nano-phase separation model, we only assume short-range interactions J(100)=−5.8 meV and J(200)=−0.85 meV. To simplify the numerical calculation we consider only the Kramer’s ground state doublet (|±>) of each Co 2+ ion. For the easy plane anisotropy of each Co 2+ ion we assume an in-plane magnetic saturation moment of and an out of plane saturation moment of . Thus, the exchange interaction H ex can be projected onto the following spin—1/2 Hamiltonian, which is of the same form as that used in ref. 15 : . Some representative N × N configurations with N =30 and N =50 were taken as the magnetic unit cell in a periodic lattice, and the spin structure and spin dynamics were calculated by the Dynamical Matrix diagonalization method [35] using the McPhase program package ( http://www.mcphase.de ). Finally, the spectra of all calculated configurations have been averaged. How to cite this article : Drees, Y. et al. Hour-glass magnetic excitations induced by nanoscopic phase separation in cobalt oxides. Nat. Commun. 5:5731 doi: 10.1038/ncomms6731 (2014).